Non-wetting droplets on hot superhydrophilic surfaces Controlling wettability by varying surface chemistry and roughness or by applying external stimuli is of interest for a wide range of applications including microfluidics, drag reduction, self-cleaning, water harvesting, anti-corrosion, anti-fogging, anti-icing and thermal management. It has been well known that droplets on textured hydrophilic, that is superhydrophilic, surfaces form thin films with near-zero contact angles. Here we report an unexpected behaviour where non-wetting droplets are formed by slightly heating superhydrophilic microstructured surfaces beyond the saturation temperature (>5 °C). Although such behaviour is generally not expected on superhydrophilic surfaces, an evaporation-induced pressure in the structured region prevents wetting. In particular, the increased thermal conductivity and decreased vapour permeability of the structured region allows this behaviour to be observed at such low temperatures. This phenomenon is distinct from the widely researched Leidenfrost and offers an expanded parametric space for fabricating surfaces with desired temperature-dependent wettability. When a water droplet is placed on a rough hydrophilic surface at room temperature, it spontaneously spreads with a near-zero contact angle ( Fig. 1a ). This behaviour is explained by the classical Wenzel equation [1] , [2] , [3] , [4] where roughness enhances the wettability of a smooth hydrophilic surface because of the reduction in the surface energy of the system. Typically, as the temperature of such surfaces increase, the wettability is expected to improve because of a decrease in the surface tension of the liquid. However, a microstructured surface heated to a critical temperature beyond the saturation temperature can sustain non-wetting droplets with contact angles as high as ≈160° ( Fig. 1b ). Detailed visualization of the solid–liquid contact line revealed that these non-wetting droplets touch the top of the pillars (inset, Fig. 1b ). 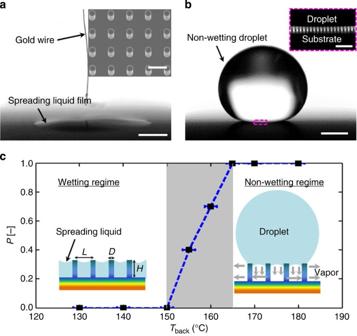Figure 1: Temperature-dependent wettability. (a) Because of roughness-enhanced wettability, a droplet deposited on a superhydrophilic surface at 120 °C spontaneously spreads into a thin film and wets the surface with a near-zero contact angle. A 25 μm diameter gold wire was used to inhibit lateral droplet movement for imaging purposes. The inset shows the scanning electron microscope image of the surface acquired at 10° inclination. Scale bars in the figure and the inset are 0.5 mm and 20 μm, respectively. (b) A similar-sized droplet at an elevated temperature of 160 °C did not wet the same surface; instead, it rests on top of the structured surface. The inset shows a magnified view of the boxed section near the droplet base indicating that the droplet remained in contact with the pillar tops. The gold wire in this case is out of the depth of field of view of the camera. Scale bars in the figure and the inset are 0.5 mm and 100 μm, respectively. (c) Probability of a non-wetting water droplet on the superhydrophilic surface as a function of substrate temperature. All droplets wet the surface when the temperature was below 150 °C, whereas all became non-wetting when the temperature was above 165 °C. The sample S1 has dimensionsD=6.6 μm,H=18.3 μm andL=20.0 μm. Figure 1: Temperature-dependent wettability. ( a ) Because of roughness-enhanced wettability, a droplet deposited on a superhydrophilic surface at 120 °C spontaneously spreads into a thin film and wets the surface with a near-zero contact angle. A 25 μm diameter gold wire was used to inhibit lateral droplet movement for imaging purposes. The inset shows the scanning electron microscope image of the surface acquired at 10° inclination. Scale bars in the figure and the inset are 0.5 mm and 20 μm, respectively. ( b ) A similar-sized droplet at an elevated temperature of 160 °C did not wet the same surface; instead, it rests on top of the structured surface. The inset shows a magnified view of the boxed section near the droplet base indicating that the droplet remained in contact with the pillar tops. The gold wire in this case is out of the depth of field of view of the camera. Scale bars in the figure and the inset are 0.5 mm and 100 μm, respectively. ( c ) Probability of a non-wetting water droplet on the superhydrophilic surface as a function of substrate temperature. All droplets wet the surface when the temperature was below 150 °C, whereas all became non-wetting when the temperature was above 165 °C. The sample S1 has dimensions D =6.6 μm, H =18.3 μm and L =20.0 μm. Full size image Although this phenomenon has not been previously reported, the effect of heating and temperature on the wetting morphology of droplets on micro-/nanostructured surfaces has been studied experimentally [5] , [6] where droplet mobility has been shown to increase with temperature. At higher temperatures, the droplets exhibit the classical Leidenfrost phenomenon [7] , [8] , where solid–liquid contact is absent because of the presence of a thin vapour layer (thickness ≈10–100 μm) [9] that completely separates the droplet from the heated surface [10] , [11] , [12] , [13] . The reported values of the Leidenfrost temperature on a flat silicon surface ranges from 200 to 390 °C [9] , [14] , [15] , [16] , [17] , [18] . Although the majority of the studies on textured surfaces report a relative increase in the Leidenfrost temperature [10] , [14] , [18] , [19] , [20] , [21] , [22] , a few recent studies reported a significant decrease in the Leidenfrost temperature on microstructured hydrophobic surfaces [23] , [24] , [25] , [26] . For example, del Cerro et al . [23] observed suspended droplets on heated surfaces composed of hydrophobic micropillars and microholes at temperatures 70% lower than the Leidenfrost point on a smooth surface. Meanwhile, Vakarelski et al . [24] reported that the Leidenfrost-like phenomenon of film boiling could be observed at extremely low superheats on superhydrophobic textured surfaces and was key to avoiding vigorous boiling because of the explosive transition from the Leidenfrost to the nucleate boiling regime. This non-wetting behaviour was attributed to the inherent water repellency of superhydrophobic surfaces, and was presumed to be absent on superhydrophilic surfaces [24] , [27] . In this work, however, we show that non-wetting droplets can reside even on superhydrophilic surfaces at superheats ( T wall − T sat ) of ≈5–50 °C, far below the Leidenfrost point, where T wall is the temperature of the substrate at the solid–liquid interface and T sat is the saturation temperature of the liquid. A mechanistic understanding of this wetting process was obtained by developing a one-dimensional force balance model, which was validated with experimental data acquired on various micropillar geometries. The low superheat that was required to obtain the non-wetting droplets on superhydrophilic surfaces is attributed to the high-pressure region created because of the presence of the micropillars that significantly increases the thermal conductivity and decreases the vapour permeability of the porous media beneath the droplet (between the droplet base and the substrate). Physical insights gained from our systematic experiments and modelling demonstrate that the wetting behaviour of droplets at room temperature does not necessarily hold at superheated conditions and, further, explain how textured hydrophilic surfaces can exhibit drastically different and yet potentially very useful wetting characteristics at superheated conditions. The observed behaviour is not only a function of the structure geometry and surface energy but also the size of the droplet and the thermal properties of the substrate material. These results have significant implications for processes such as spray cooling of hot metals during metallurgical processes, cooling of nuclear reactors during emergency shutdown, heat exchangers and cooling of overheated components in high-power-density thermal applications [12] where solid–liquid contact is desired for improved heat transfer performance. The non-wetting mechanism also suggests a route to sustained surface-energy-independent drag reducing surfaces at superheats significantly lower than the Leidenfrost point [25] . Experiments Well-defined silicon micropillar arrays arranged in a square pattern with varying diameter ( D ), height ( H ) and pitch ( L; see Table 1 ) were fabricated using standard contact photolithography and deep reactive ion etching. The scanning electron microscope images of the six test samples used in this investigation are shown in the Supplementary Fig. S1 . The typical intrinsic contact angle ( θ Y ) of organically contaminated SiO 2 surfaces is ≈38–42° (refs 28 , 29 , 30 ), which was also confirmed in our experiments. A platinum resistive heater and four sensors for measuring temperature were patterned on the backside of the sample using e-beam evaporation and standard lift-off processes. The details of the microfabrication, sample cleaning procedure, experimental set-up and methodology are discussed in the Methods section. Table 1 Test sample dimensions. Full size table We performed droplet wetting experiments on superheated hydrophilic microstructured surfaces at atmospheric pressure to investigate the effect of substrate temperature, surface geometry ( D , H and L ) and droplet size on wetting morphology. To determine the critical deposition temperature beyond which droplets become non-wetting, droplets were gently deposited onto the microstructured surface at a prescribed temperature. Figure 1c summarizes the probability, P , of obtaining non-wetting water droplets (out of 10 attempts) on the superhydrophilic surface as a function of the back side substrate temperature. All droplets wetted the surface ( P =0) when the substrate temperature was <150 °C, whereas none of them wetted ( P =1) when the temperature was >165 °C. To investigate the effect of droplet size on the wetting state, experiments were also carried out where the substrate temperature was lowered and allowed to stabilize after depositing a non-wetting droplet. Details of a typical experiment are shown in Fig. 2 . 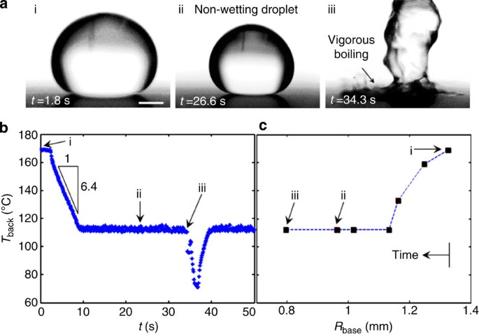Figure 2: Wetting transition. (a) Time-lapse images of a droplet on a superhydrophilic surface. Images were acquired (i) after droplet deposition (t=1.8 s), (ii) before wetting at the lower steady-state temperature (t=26.6 s), and (iii) after wetting, which led to vigorous boiling (t=34.3 s). Scale bar, 1 mm. (b) Corresponding substrate temperature as a function of time. The droplet was deposited at 170 °C att=0 s (i) and subsequently the substrate temperature was reduced at a rate of ≈6 °C s−1to 112 °C in ≈9 s (ii). The droplet continued to evaporate (and the receding contact angle changed with time) until transition to the wetted state att=34.3 s (iii) as indicated by the sudden reduction in substrate temperature. (c) Relationship between the substrate temperature and the base radius of an evaporating droplet measured (solid black square symbols) from the time-lapse images. The droplet transitioned at a base radius of 0.80 mm. The sample S1 has dimensionsD=6.6 μm,H=18.3 μm andL=20.0 μm. Figure 2ai corresponds to a newly deposited non-wetting water droplet on a superhydrophilic surface at a temperature of 170 °C ( Fig. 2b ). Once deposited, the droplet remained non-wetting ( Fig. 2aii ) even after the temperature was subsequently reduced and stabilized at 112 °C ( Fig. 2b ). It is noteworthy that this surface temperature (112 °C) was significantly lower than the critical transition temperature shown in Fig. 1c . When sufficient time was given for the droplet to evaporate, however, a spontaneous wetting transition followed by vigorous nucleate boiling occurred at t =34.3 s ( Fig. 2aiii ) corresponding to a droplet base radius of R base ≈0.80 mm ( Fig. 2c ). Because of the increased solid–liquid contact following transition, we observed a significant temperature reduction in the substrate beneath the droplet ( Fig. 2b ). A movie illustrating the dynamic nature of the non-wetting droplet corresponding to the data in Fig. 2 can be found in the Supplementary Movie 1 . Figure 2: Wetting transition. ( a ) Time-lapse images of a droplet on a superhydrophilic surface. Images were acquired (i) after droplet deposition ( t =1.8 s), (ii) before wetting at the lower steady-state temperature ( t =26.6 s), and (iii) after wetting, which led to vigorous boiling ( t =34.3 s). Scale bar, 1 mm. ( b ) Corresponding substrate temperature as a function of time. The droplet was deposited at 170 °C at t =0 s (i) and subsequently the substrate temperature was reduced at a rate of ≈6 °C s −1 to 112 °C in ≈9 s (ii). The droplet continued to evaporate (and the receding contact angle changed with time) until transition to the wetted state at t =34.3 s (iii) as indicated by the sudden reduction in substrate temperature. ( c ) Relationship between the substrate temperature and the base radius of an evaporating droplet measured (solid black square symbols) from the time-lapse images. The droplet transitioned at a base radius of 0.80 mm. The sample S1 has dimensions D =6.6 μm, H =18.3 μm and L =20.0 μm. Full size image Modelling To explain the mechanism of non-wetting droplets on a superhydrophilic surface, we developed a one-dimensional force balance model that includes gravity and surface tension as the wetting forces and evaporation-induced pressure as the non-wetting force. We attribute the higher superheat required for initial droplet deposition ( t =0 s, Fig. 2b ) compared with that necessary to maintain the non-wetting droplet ( t >9 s, Fig. 2b ) to the additional wetting forces of water hammer [31] , [32] , [33] and dynamic pressure at the start of the experiment. Consequently, the non-wetting force and hence the temperature necessary to sustain a non-wetting droplet was lower compared with that needed to initially deposit a non-wetting droplet. The liquid–vapor interface in our experiments is concave outwards and surface tension acts in the same direction as gravity for a superhydrophilic surface ( Fig. 3a,b ). It is noteworthy that for a typical superhydrophobic surface, the curvature of the liquid–vapor interface is concave inwards counteracting wetting [34] . The local wetting force acting around each pillar, f W = πD ϒ LV , shown schematically in Fig. 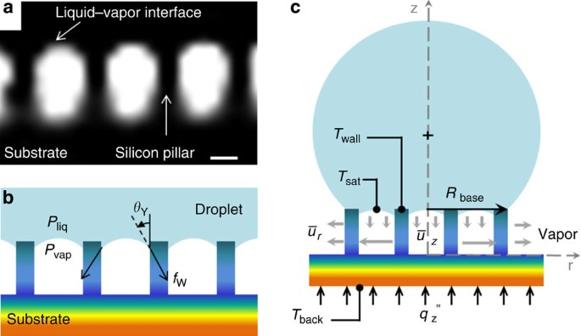Figure 3: Wetting mechanism. (a) A magnified image of the contact between the droplet base and the pillar tops. The droplet touches the side walls of the pillar locally exhibiting the intrinsic contact angle (<90°, hydrophilic), and the meniscus shape at the liquid–vapor interface is concave outwards. The high pressure beneath the droplet (Pvap>Pliq>Pamb) maintains the droplet in this composite state and enables the visualization of the meniscus shape. This curvature is apparent from the captured image where the evaporation-induced high pressure provided an external anti-wetting force that maintained the droplet in a composite state for visualization. Scale bar, 10 μm. (b) Schematic showing the outward curvature of the liquid–vapor interface (not to scale). Because of the hydrophilicity, the vertical component of the surface tension force acts downwards to induce wetting. (c) Schematic of a non-wetting evaporating droplet resting on a microstructured hydrophilic surface (not to scale). Heat is conducted through the substrate and primarily through the pillars to induce evaporation at the liquid–vapor interface, which is assumed to be at saturation temperatureTsat≈100 °C. Continuous supply of vapour to the porous mediaviaevaporation creates a high-pressure region beneath the droplet. The pressure difference drives the vapor radially outwards. The vapour thickness was assumed to be the same as the pillar height. 3b , can be used to calculate the global average wetting force, F W , acting on the droplet as Figure 3: Wetting mechanism. ( a ) A magnified image of the contact between the droplet base and the pillar tops. The droplet touches the side walls of the pillar locally exhibiting the intrinsic contact angle (<90°, hydrophilic), and the meniscus shape at the liquid–vapor interface is concave outwards. The high pressure beneath the droplet ( P vap > P liq > P amb ) maintains the droplet in this composite state and enables the visualization of the meniscus shape. This curvature is apparent from the captured image where the evaporation-induced high pressure provided an external anti-wetting force that maintained the droplet in a composite state for visualization. Scale bar, 10 μm. ( b ) Schematic showing the outward curvature of the liquid–vapor interface (not to scale). Because of the hydrophilicity, the vertical component of the surface tension force acts downwards to induce wetting. ( c ) Schematic of a non-wetting evaporating droplet resting on a microstructured hydrophilic surface (not to scale). Heat is conducted through the substrate and primarily through the pillars to induce evaporation at the liquid–vapor interface, which is assumed to be at saturation temperature T sat ≈100 °C. Continuous supply of vapour to the porous media via evaporation creates a high-pressure region beneath the droplet. The pressure difference drives the vapor radially outwards. The vapour thickness was assumed to be the same as the pillar height. Full size image where πR base 2 / L 2 accounts for the number of pillars in contact with the droplet base area, and ϒ LV is the interfacial liquid–vapor surface tension of water at 100 °C. The experimentally measured global apparent contact angle of the evaporating droplet on the structured surface varied between ≈130° and ≈160°. The observed change in the apparent contact angle was because of a combination of the highly dynamic nature of the evaporating droplet ( Supplementary Movie 1 ) and the decrease in the effect of gravity with the continuous decrease in size, rendering the models (for example, Cassie) in literature for predicting contact angle of a composite droplet invalid. As a result, we decoupled our analysis from the apparent contact angle of the droplet and accordingly used the experimentally measured droplet base radius to calculate the wetting force. Gravity was neglected in this calculation because of the relatively large contribution of the surface tension force compared with the weight of the droplet. For the experimental data discussed in this paper, the surface tension force was approximately an order of magnitude larger than the weight of the droplet. The force due to the 25 μm hydrophobized gold wire that was used to hold the droplet in position to avoid lateral movement (see Fig. 1a ) was even smaller justifying the use of equation (1). The high-pressure vapour cushion beneath the droplet provides the non-wetting force. This force is fundamentally similar to the non-wetting force in a Leidenfrost phenomenon on a flat surface; however, the homogenous vapour cushion is replaced by a porous media in our case. As shown schematically in Fig. 3c , heat conducts through the substrate and then primarily through the silicon pillars to induce evaporation at the liquid–vapor interface. The detailed modelling of the overall thermal resistance from the backside of the substrate to the liquid–vapor interface is shown in the Supplementary Information . The evaporation from the droplet spherical cap is negligible when compared with that at the droplet base [35] . Assuming uniform evaporation from the droplet base we then related the conducted heat with the latent heat of vaporization of water to estimate the normal mean velocity ū z of the vapour leaving the liquid–vapour interface at the droplet base (see Fig. 3c ) as follows: where T back is the backside temperature, ρ vap and h fg are the density of vapour and the latent heat of vaporization of water, respectively, A c is the area of a unit cell ( A c = L 2 ) and R th is the overall thermal resistance in units of K W −1 (see Supplementary Note 1 ). As H / R base <<1, the mean velocity in the z -direction ū z is small compared with the mean velocity in the radial direction ū r (that is ū z / ū r <<1) allowing us to apply the lubrication approximation. The continuity equation at any radial position r can then be written as Substituting equation (2) into equation (3) gives a relationship between the average radial velocity and overall temperature difference ( T back − T sat ) as Next, we solve the appropriate momentum equation for flow in porous media, which in this case can be reduced to the classical Brinkman equation [36] , [37] , where ε is the porosity given by ε =1− πD 2 / L 2 , K is the permeability of the porous media [38] , μ vap is the absolute viscosity of vapour and P vap ( r ) is the vapour pressure at a radial position r from the droplet centerline. Equation (5) was solved by imposing the no-slip boundary conditions ( u =0) at the pillar base ( z =0) and pillar top ( z = H ) to obtain the velocity profile of the vapour beneath the droplet base, which was then integrated from the pillar base to the pillar top to obtain the mean radial velocity as follows: where and has units of m −1 . The mean radial velocity obtained from conservation of energy (equation (4)) and from conservation of momentum (equation (6)) were then equated to solve for the radial gauge pressure profile as where P amb is the ambient pressure (≈101.3 kPa) at the edge of the droplet. The non-wetting force, can now be obtained by integrating the gauge pressure from equation (7) over the base area of the droplet and is given by The criteria for the wetting transition reported in Fig. 2b was then estimated by equating the two competing forces (equation (1) and equation (8)) and solving for the superheat using the thermal resistance network as follows: where R evap and R s are the evaporation [12] and spreading thermal resistances (see Supplementary Note 1 ). All thermophysical properties were evaluated at 100 °C. It is noteworthy that the backside temperature T back that was measured experimentally is dependent on the substrate thickness and was not an appropriate measure of the superheat. Referring to the thermal resistance network in Supplementary Fig. S4 , the superheat ( T wall − T sat ), which is independent of substrate thickness was accordingly obtained by multiplying ( T back − T sat ) by the appropriate resistance ratio ( R s + R evap )/ R th . The first term in parenthesis on the right hand side of equation (9) comprises fluid properties, which equivalently represents an apparent heat flux term (Wm −2 ). The second term in parenthesis, which is dependent on the geometry of the textured surface and the thermal conductivity of the material, represents an effective thermal resistance (m 2 K W −1 ). The third non-dimensional term, which originated from the Brinkman equation accounts for the viscous losses incurred by the presence of the micropillars. Validation We used our model to explain the effect of droplet size and microstructure geometry on the transition superheat. Despite the simple one-dimensional force balance adopted to obtain equation (9), Fig. 4 shows reasonable agreement between the experimental data and the model prediction over the wide parametric space investigated in this study. In addition, experiments carried out on various geometries (samples S2–S6; see Table 1 ) confirmed that the superheat required to suspend a non-wetting droplet on textured hydrophilic surfaces decreases when D increases ( Fig. 4b ), and when H and L decrease ( Fig. 4c,d , respectively). The shift in the transition curve was less sensitive to the contact angles for the range of intrinsic wettability investigated in this study (see Supplementary Note 2 ). 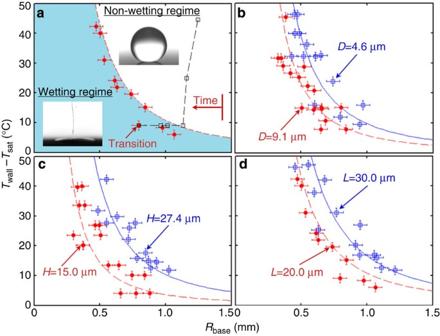Figure 4: Validation and parametric effects. Mechanistic understanding from model and experimental results show the effect of micropillar geometry on transition superheat. (a) Experimentally observed transition points (red solid circle) and model prediction (red dashed line) for test sample S1 with dimensionsD=6.6 μm,H=18.3 μm andL=20.0 μm show good agreement. The red dashed line, which was obtained from equation (9), separates the wetting from the non-wetting regime. The black squares correspond to the continuously evaporating non-wetting droplet inFig. 2(right to left as indicated by the time axis). The droplet transitioned to a thin film on entering the wetting regime and the last point before transition represents a sample transition data indicated by a red solid circle. All other transition data points were obtained using similar analysis methodology. Experimental data and model prediction of superheat as a function of base radius demonstrate the effect of (b) diameterDfor S2 and S3, (c) heightHfor S4 and S5, (d) pitchLfor S1 and S6. Note that the wall temperature (Twall) was deduced from the experimentally measured backside temperature (Tback) using a thermal resistance network shown in the Supplementary. An intrinsic contact angle of 42° was used for these calculations. The error bars for the superheat were obtained from the s.d. of superheat versus time plot of 20 randomly selected experiments, whereas the error bars for the base radius of the droplet were obtained from the s.d. of 10 randomly selected experiments by repeatedly (10 times each) calculating the base radius from the captured images. Figure 4 also shows that the superheat at transition is inversely proportional to the square of the base radius of the droplet. This result can be explained by the force balance, where calculations show that the wetting and the non-wetting forces scale as R base 2 (equation (1)) and R base 4 (equation (8)), respectively. Accordingly, the superheat that is obtained by equating the two competing forces scales as . This inverse quadratic dependence of the superheat on the base radius of the evaporating droplet indicates that smaller droplets require higher superheat to remain non-wetting, which is consistent with the experiments. Figure 4: Validation and parametric effects. Mechanistic understanding from model and experimental results show the effect of micropillar geometry on transition superheat. ( a ) Experimentally observed transition points (red solid circle) and model prediction (red dashed line) for test sample S1 with dimensions D =6.6 μm, H =18.3 μm and L =20.0 μm show good agreement. The red dashed line, which was obtained from equation (9), separates the wetting from the non-wetting regime. The black squares correspond to the continuously evaporating non-wetting droplet in Fig. 2 (right to left as indicated by the time axis). The droplet transitioned to a thin film on entering the wetting regime and the last point before transition represents a sample transition data indicated by a red solid circle. All other transition data points were obtained using similar analysis methodology. Experimental data and model prediction of superheat as a function of base radius demonstrate the effect of ( b ) diameter D for S2 and S3, ( c ) height H for S4 and S5, ( d ) pitch L for S1 and S6. Note that the wall temperature ( T wall ) was deduced from the experimentally measured backside temperature ( T back ) using a thermal resistance network shown in the Supplementary. An intrinsic contact angle of 42° was used for these calculations. The error bars for the superheat were obtained from the s.d. of superheat versus time plot of 20 randomly selected experiments, whereas the error bars for the base radius of the droplet were obtained from the s.d. of 10 randomly selected experiments by repeatedly (10 times each) calculating the base radius from the captured images. Full size image The developed model provides the following physical insight into the mechanism of the wetting transition. When compared with Leidenfrost, the high thermal conductivity of the microstructured porous media increases the effective thermal conductivity of the gap between the droplet and the substrate, leading to increased evaporation rates at lower superheat. This effect in combination with the decreased vapour permeability due to viscous losses from the side walls of the micropillars significantly increases the pressure of the vapour cushion beneath the droplet base. As a result, the non-wetting force in our experiments was significantly higher and transition was observed at superheats significantly lower than those required for the classical Leidenfrost phenomenon. Further, the vapour layer thickness based on the classical Leidenfrost model for porous media by Avedisian et al . [10] was estimated to be ≈20 μm for our experimental conditions. This estimation of the gap between the droplet base and pillar top should have been apparent in the inset image in Figs 1b and 3a where the 20-μm gap between neighbouring pillars is visible. Accordingly, the non-wetting droplets in our experiments are distinct from the classical Leidenfrost phenomenon where solid–liquid contact is completely absent because of the presence of a vapour layer that separates the droplet from the heated surface. The understanding gained from this study suggests that low solid fraction, but high aspect ratio, small-scale structures with low thermal conductivities should be used to extend the transition superheat for heat transfer applications such as spray cooling of hot metals, cooling of nuclear reactors during emergency shutdown, heat exchangers and cooling of overheated components in high-power-density thermal applications. Conversely, larger-scale feature sizes and high thermal conductivity structures are desirable in applications where contact of the heated surface should be minimized to reduce corrosion or to generate a stable vapour on nominally hydrophilic surfaces upon mild heating for hydrodynamic drag reduction, thus opening a range of potential material systems for these applications. In addition, this framework can be extended to investigate the effect of geometry and material properties for the design of superhydrophobic surfaces at elevated temperatures. Microfabrication Standard contact photolithography and deep reactive ion etching were used to create silicon micropillars in a square pattern on the front side. Scanning electron microscope images of the six test samples used in this study is shown in Supplementary Fig. S1 . A thin-film resistive heater and temperature sensors were patterned on the backside of the test sample using e-beam evaporation (100 nm platinum on top of a 20 nm titanium adhesive layer) and acetone lift-off. An image of a typical test sample after the microfabrication process was complete is shown in Supplementary Fig. S2 . The sensors were calibrated in a conventional oven using a commercial platinum resistance temperature detector with a National Institute of Standards and Technology-traceable calibration prior to experiment. The resistance versus temperature data of the sensors was linear with <1% root mean square error. Experimental set-up The experimental set-up is shown in Supplementary Fig. S3 . A pipette (b) was used to gently dispense droplets onto the textured surface, which was mounted on a three-dimensional stage (g) and heated using a direct current power source (c). Images were captured using CMOS camera (Phantom V7.1, Vision Research; a), whereas the backside temperature was acquired using a DAQcard (USB-6251, National Instruments; e). As discussed in Fig. 2 , the substrate temperature was lowered and allowed to stabilize after depositing a non-wetting droplet on the superhydrophilic surface. The initial high temperature, which was necessary to overcome transient effects such as water hammer, was obtained by directly heating the sample through circuit 3-4-5-6-7 (solid line), whereas the lower steady-state temperature was established by actively controlling the heating power using a three-way switch (d) and a solid-state relay (f) through circuit 3-4-8-9-10-6-7 (broken line), which opens and closes at junction 9-10 based on the temperature feedback from the sensors. The turning on and off of the circuit at junction 9-10 was used to establish the lower steady-state temperature (>9 s; Fig. 2b ). Experiment methodology A standard sample cleaning procedure was developed before experiments, where each sample was cleaned with acetone, methanol, isopropanol and deionized water, dried with nitrogen gas and oxygen plasma treated (Harrick Plasma) for 30 min. Reagent grade water (Sigma-Aldrich, CAS: 7732-18-5) was used as the working fluid. The sample was then allowed to relax in the laboratory environment such that it recovered the intrinsic static contact angle of ≈38–42° (refs 28 , 29 , 30 ) under ambient conditions. The advancing contact angle was ≈40–42°, whereas the receding contact angle was ≈9–12° (ref. 39 ). Droplets were dispensed onto the heated surface whose temperature was monitored and recorded using a data acquisition system. A 25 μm diameter gold wire, functionalized with a 1 mM ethanol solution of 1H, 1H, 2H, 2H-perfluorodecanethiol (Sigma-Aldrich), was used to prevent lateral motion of the droplet outside of the imaging camera’s field of view. How to cite this article: Adera, S. et al . Non-wetting droplets on hot superhydrophilic surfaces. Nat. Commun. 4:2518 doi: 10.1038/ncomms3518 (2013).